WheatMds-1encodes a heat-shock protein and governs susceptibility towards the Hessian fly gall midge Gall midges induce formation of host nutritive cells and alter plant metabolism to utilize host resources. Here we show that the gene Mayetiola destructor susceptibility-1 on wheat chromosome 3AS encodes a small heat-shock protein and is a major susceptibility gene for infestation of wheat by the gall midge M. destructor , commonly known as the Hessian fly. Transcription of Mayetiola destructor susceptibility-1 and its homoeologs increases upon insect infestation. Ectopic expression of Mayetiola destructor susceptibility-1 or induction by heat shock suppresses resistance of wheat mediated by the resistance gene H13 to Hessian fly. Silencing of Mayetiola destructor susceptibility-1 by RNA interference confers immunity to all Hessian fly biotypes on normally susceptible wheat genotypes. Mayetiola destructor susceptibility-1 -silenced plants also show reduced lesion formation due to infection by the powdery mildew fungus Blumeria graminis f. sp. tritici . Modification of susceptibility genes may provide broad and durable sources of resistance to Hessian fly, B. graminis f. sp. tritici , and other pests. Plant parasites, including many insects, nematodes, and microbes manipulate plants to utilize host resources. Hessian fly, a member of a large group of gall-inducing insects called gall midges, is a destructive insect pest of wheat, and a model organism to study plant–insect interactions [1] , [2] . Hessian fly larvae live between leaf-sheaths near the base of wheat seedlings. Even though it does not induce the formation of a typical outgrowth gall, a Hessian fly larva is able to convert the whole susceptible plant into a gall by inducing the formation of nutritive cells at the feeding site and by inhibiting plant growth while maintaining the infested plant alive as a source for nutrients [2] , [3] . The infested susceptible plant dies eventually after the insect ceases feeding on the plant. Successful infestation is accompanied by increased epidermal permeability of sheath cells, an indicator of nutritive cell formation [4] . Hessian fly larvae also suppress plant defence and reprogram metabolic pathways of susceptible plants during compatible interactions [5] . In plants carrying a resistance (R) gene directed against Hessian fly infestation, a larva is unable to establish a permanent feeding site and dies within 3–5 days after hatching. Resistant plants resume normal growth after some initial growth deficit [6] . Thirty-two major R genes to Hessian fly have been identified in wheat or wheat relatives [7] . All known R genes have a typical gene-for-gene relationship with Hessian fly avirulence as observed in many plant–pathogen systems. Many R genes have been deployed to the field and are initially highly effective in protecting wheat from Hessian fly damage [1] , [2] . However, resistance mediated by R genes is short-lived and usually overcome by the insect within 3–6 years after the deployment of a resistant cultivar due to the appearance of new virulent Hessian fly biotypes [8] . All known R genes in wheat are also temperature sensitive and lose resistance to Hessian fly above 28 °C (ref. 9 ). Further insights into the molecular aspects of the wheat–Hessian fly interaction are therefore needed to improve wheat resistance. Expression profiling of nearly isogenic susceptible and resistant wheat cultivars revealed that many host genes are up- or downregulated following Hessian fly infestation [5] . On the basis of the gene annotation, the changes in susceptible wheat are consistent with the conversion of the sheath cells to a nutrient sink with concomitant increases in carbohydrate metabolism, amino-acid biosynthesis and nutrient transport. The changes in gene expression in susceptible plants are also consistent with the dramatic shift from carbon-containing compounds to nitrogen-containing compounds that occurs during compatible interactions [10] . Some of the specifically induced genes with the greatest expression are predicted to be involved in stress responses, likely as the consequence of developmentally inappropriate alteration to host cell physiology or the hijacking of the stress responses for the benefit of Hessian fly larvae [5] . Here, we present a functional analysis of a predicted heat-shock protein (HSP) gene that was represented by the EST CD453475, named here Mayetiola destructor susceptibility gene-1 ( Mds-1 ). Mds-1 gene showed the highest level of induction in wheat seedlings during compatible interactions to Hessian fly infestation [5] . We examined the impact of silencing and ectopic expression of Mds-1 in susceptible and resistant wheat genotypes, respectively, on Hessian fly larval survival and development. Hessian fly infection induces Mds-1 On the basis of the EST CD453475 sequence, a full-length cDNA and the gene (GenBank Accession Code JN162442) were cloned from the susceptible wheat Newton by RACE-PCR and PCR ( Supplementary Fig. S1 ). Mds-1 encodes a protein of 151 amino-acid residues and has 96% identity with a previously characterized HSP, HSP16.9, a member of a group of proteins with the α-crystallin domain [11] ( Fig. 1a ). Without infestation, very low levels of Mds-1 transcript were detected in wheat leaf-sheaths ( Fig. 1b ), the feeding site for Hessian fly larvae. Higher transcript levels were found in developing grains. Both the transcript and protein levels increased in plants during compatible interactions following Hessian fly infestation, but no apparent increase in the transcript or protein levels was observed in plants during incompatible interaction with the wheat cultivar Molly ( Fig. 1c ), which carries the R gene H13 (ref. 12 ). 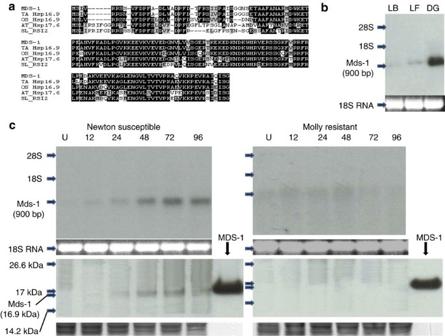Figure 1:Mds-1encodes a small heat-shock protein induced by Hessian fly. (a) An alignment of MDS-1 and related proteins from various plant species. The Genbank accession codes for the proteins are as follows: TA_Hsp16.9 (1GME_A); OS_Hsp16.9 (P27777); AT_Hsp17.6 (CAA34208); and SL_RSI2 (AF123255). TA, OS, AT and SL representTriticum aestivum,Oryza sativa,Arabidopsis thalianaandSolanum lycopersicum, respectively.Mds-1was cloned from the susceptible wheat cultivar Newton. (b)Mds-1transcript levels in uninfested susceptible Newton wheat leaf blades (LB), leaf-sheaths (LF) and developing grains (DG). 28S, 18S and Mds-1 (900 bp) along with arrows on the left of the northern blot represent the locations of 28 S rRNA, 18 S rRNA andMds-1mRNA. An 18S rRNA image of the gel is given below the blot as loading control. (c)Mds-1is upregulated during Hessian fly infestation in susceptible Newton, but not in resistant Molly wheat. Northern (upper panels) and western (lower panel) blot analyses ofMds-1transcript and protein with samples from susceptible Newton plants (left panels) and resistant Molly plants (right panels) at 0 (U), 12–96 h, respectively, after infestation with Hessian fly biotypeGP. Plants were infested by confining mated females in pots with screens. Females deposit eggs on leaf blades. Neonates migrate into a plant and live between leaf-sheaths next to the base. The time point 0 was taken right before neonates reach the feeding site. 28S, 18S, Mds-1 (900 bp) and 18S rRNA are as described inb. The positions of protein size markers and the location of the Mds-1 protein are given on the left of the western blots along with arrows. MDS-1 represents a recombinant protein control (0.116 μg per lane). A coomassie-blue gel image is given under each western blot as loading control. Figure 1: Mds-1 encodes a small heat-shock protein induced by Hessian fly. ( a ) An alignment of MDS-1 and related proteins from various plant species. The Genbank accession codes for the proteins are as follows: TA_Hsp16.9 (1GME_A); OS_Hsp16.9 (P27777); AT_Hsp17.6 (CAA34208); and SL_RSI2 (AF123255). TA, OS, AT and SL represent Triticum aestivum , Oryza sativa , Arabidopsis thaliana and Solanum lycopersicum , respectively. Mds-1 was cloned from the susceptible wheat cultivar Newton. ( b ) Mds-1 transcript levels in uninfested susceptible Newton wheat leaf blades (LB), leaf-sheaths (LF) and developing grains (DG). 28S, 18S and Mds-1 (900 bp) along with arrows on the left of the northern blot represent the locations of 28 S rRNA, 18 S rRNA and Mds-1 mRNA. An 18S rRNA image of the gel is given below the blot as loading control. ( c ) Mds-1 is upregulated during Hessian fly infestation in susceptible Newton, but not in resistant Molly wheat. Northern (upper panels) and western (lower panel) blot analyses of Mds-1 transcript and protein with samples from susceptible Newton plants (left panels) and resistant Molly plants (right panels) at 0 (U), 12–96 h, respectively, after infestation with Hessian fly biotype GP . Plants were infested by confining mated females in pots with screens. Females deposit eggs on leaf blades. Neonates migrate into a plant and live between leaf-sheaths next to the base. The time point 0 was taken right before neonates reach the feeding site. 28S, 18S, Mds-1 (900 bp) and 18S rRNA are as described in b . The positions of protein size markers and the location of the Mds-1 protein are given on the left of the western blots along with arrows. MDS-1 represents a recombinant protein control (0.116 μg per lane). A coomassie-blue gel image is given under each western blot as loading control. Full size image Silencing of Mds-1 inhibits Hessian fly development Expression of Mds-1 was reduced by virus-induced gene silencing (VIGS) [13] to determine the requirement for Mds-1 expression during Hessian fly infestation. VIGS treatment of seedlings of the susceptible wheat Newton prevented the induction of Mds-1 in Hessian fly-infested plants and rendered the susceptible genotype immune to Hessian fly infestation ( Fig. 2a ). Seven Hessian fly populations representing at least 30 biotypes were tested, and all biotypes were incompatible on Mds-1- silenced wheat seedlings ( Supplementary Table S1 ). The effect of Mds-1 silencing was also assessed in stable transgenic plants. Twenty-four independent transgenic lines of the wheat cultivar Bobwhite, a Spring wheat with high efficiency for genetic transformation, were generated with a construct expressing double-stranded RNA for Mds-1 silencing. Twenty of the transformants showed suppression of Mds-1 induction by Hessian fly, whereas the remaining four did not have the suppression effect ( Supplementary Table S2 ). The transgenic plants and their progeny with suppressed Mds-1 lost susceptibility to Hessian fly biotype GP ( Fig. 2b , Supplementary Table S2 , Supplementary Fig. S4 ). Transgenic lines T1630, T1639, T2095 and T2357 were advanced to T2 generation (equivalent to F2 offspring from F0), and all these transgenic lines were resistant to all biotypes tested so far ( Supplementary Table S1 ). 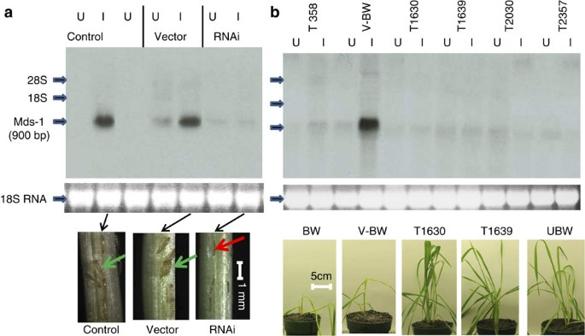Figure 2: Silencing ofMds-1in wheat confers immunity to susceptible plants. (a) Transient silencing ofMds-1in the susceptible genotype Newton confers immunity to Hessian fly biotypeGP. Newton is a winter wheat and the susceptible recipient parents of several isogenic lines including Molly and Iris that contain different R genes12. Northern blot analysis ofMds-1transcript in plants of untreated control, treated with the original virus (Vector) or treated with the modified virus that carried the 338-bp fragment ofMds-1(RNAi) (Supplementary Fig. S2a). U, uninfested; I, infested plants. 28S, 18S and Mds-1 (900 bp) along with arrows on the left of the northern blot represent the locations of 28S rRNA, 18S rRNA andMds-1mRNA. An 18S rRNA image is given under the blot as loading control. Phenotypes of Hessian fly larvae on the control, vector- and RNAi-treated plants are given in the lower panel. Green arrows point to live larvae, the red arrow points to a dead larva. (b) Suppression ofMds-1expression in transgenic Bobwhite plants confers immunity to Hessian fly biotypeGPinfestation. Bobwhite is a spring wheat line with high efficiency for genetic transformation. Bobwhite is susceptible to Hessian fly infestation. The upper panel is a northern blot of independent transgenic Bobwhite lines T385, T1630, T1639, T2030, T2357, produced with an RNAi construct (Supplementary Fig. S2b); and an empty vector-transformed Bobwhite wheat, V-BW, with (I) and without (U) Hessian fly infestation. Other denotations are the same as ina. The lower panel shows phenotypic differences among a non-transgenic Bobwhite plant (BW), an empty vector-transgenic plant (V-BW) and theMds-1-silenced plants T1630 and T1639 after Hessian fly infestation. Growth of infested BW and V-BW was inhibited, but growth of infested T1630 and T1639 plants was comparable to that of uninfested control Bobwhite (UBW) plants. Resistance was observed in both seedling and adult transgenic plants. Figure 2: Silencing of Mds-1 in wheat confers immunity to susceptible plants. ( a ) Transient silencing of Mds-1 in the susceptible genotype Newton confers immunity to Hessian fly biotype GP . Newton is a winter wheat and the susceptible recipient parents of several isogenic lines including Molly and Iris that contain different R genes [12] . Northern blot analysis of Mds-1 transcript in plants of untreated control, treated with the original virus (Vector) or treated with the modified virus that carried the 338-bp fragment of Mds-1 (RNAi) ( Supplementary Fig. S2a ). U, uninfested; I, infested plants. 28S, 18S and Mds-1 (900 bp) along with arrows on the left of the northern blot represent the locations of 28S rRNA, 18S rRNA and Mds-1 mRNA. An 18S rRNA image is given under the blot as loading control. Phenotypes of Hessian fly larvae on the control, vector- and RNAi-treated plants are given in the lower panel. Green arrows point to live larvae, the red arrow points to a dead larva. ( b ) Suppression of Mds-1 expression in transgenic Bobwhite plants confers immunity to Hessian fly biotype GP infestation. Bobwhite is a spring wheat line with high efficiency for genetic transformation. Bobwhite is susceptible to Hessian fly infestation. The upper panel is a northern blot of independent transgenic Bobwhite lines T385, T1630, T1639, T2030, T2357, produced with an RNAi construct ( Supplementary Fig. S2b ); and an empty vector-transformed Bobwhite wheat, V-BW, with (I) and without (U) Hessian fly infestation. Other denotations are the same as in a . The lower panel shows phenotypic differences among a non-transgenic Bobwhite plant (BW), an empty vector-transgenic plant (V-BW) and the Mds-1 -silenced plants T1630 and T1639 after Hessian fly infestation. Growth of infested BW and V-BW was inhibited, but growth of infested T1630 and T1639 plants was comparable to that of uninfested control Bobwhite (UBW) plants. Resistance was observed in both seedling and adult transgenic plants. Full size image Mds-1 confers resistance gene plants susceptibility Owing to the hexaploid nature, a wheat gene usually has at least three homoeologs from A, B and D genomes that share high nucleotide sequence similarity. RNA interference (RNAi) in transgenic and VIGS-treated plants may have reduced the abundance of Mds-1 and related transcripts. The silencing strategy did concomitantly reduce levels of Mds-1 -related transcripts ( Supplementary Figs S5a,b and S6 ). To determine whether Mds-1 homoeologs are involved in wheat susceptibility to Hessian fly, we mapped Mds-1 to wheat chromosome 3AS using Chinese Spring wheat ditelosomic and deletion lines ( Supplementary Fig. S7a1,a2 and b ) [14] . The homoeologs of Mds-1 on chromosomes 3B and 3D were identified by searching genomic sequences derived from these two chromosomes specifically ( Supplementary Fig. S8 ) [15] , [16] . The two homoeolous genes on B and D genomes, named as HB and HD, respectively, were mapped to the similar distal regions of chromosomal 3B and 3DS using gene-specific primer pairs ( Supplementary Figs S7a3,a4,b and S8 ). Transcript abundance of all these three homoeologs was induced by Hessian fly infestation and by heat stress ( Supplementary Fig. S7c,d ). The ditelosomic lines of Chinese Spring wheat missing Mds-1 or either one of its two homoeologs on B and D chromosomes are still susceptible to Hessian fly infestation, indicating that each of the homoeologous genes is able to confer wheat susceptibility to Hessian fly infestation. To determine whether Mds-1 expression alone is sufficient for wheat susceptibility to Hessian fly, we took advantage of the lack of induction of Mds-1 by Hessian fly in the resistant wheat cultivar Molly. Mds-1 was ectopically expressed at high levels in Molly through stable transformation ( Supplementary Fig. S9 ). Although normally resistant to Hessian fly, Molly plants became susceptible to the insect when Mds-1 was ectopically expressed ( Fig. 3a ). Seven independent transgenic lines with ectopic Mds-1 expression were produced to avoid positional or other undesirable effects ( Supplementary Table S2 ). All seven transgenic lines with ectopic Mds-1 expression were susceptible to Hessian fly infestation. In addition to ectopic expression, heat stress was also adapted to induce Mds-1 expression as Mds-1 encodes a HSP. When Molly seedlings were stressed at 37 °C and then allowed to recover at 20 °C, high levels of Mds-1 transcript were observed ( Fig. 3b ), and the plants with high levels of Mds-1 expression became susceptible ( Fig. 3c ). Heat-shock studies with wheat cultivars containing other R genes gave similar results ( Supplementary Fig. S10 ). Heat-induced wheat susceptibility was not due to a general stress response as susceptibility did not occur in Mds-1 -silenced, transgenic plants ( Fig. 4 ). 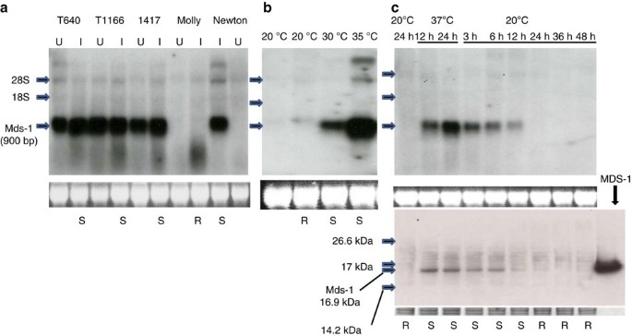Figure 3: Ectopic expression and heat induction ofMds-1in resistant wheat. (a) Ectopic expression ofMds-1correlates with a phenotype switch of Molly plants from resistance to susceptibility to Hessian fly biotypeGPinfestation. Northern blot analysis ofMds-1transcript in samples from transgenic Molly lines T640, T1166 and T1417 (Supplementary Table S2,Supplementary Fig. S9); non-transgenic, resistant Molly; and the susceptible wheat Newton with (I) and without (U) Hessian fly (biotypeGP) infestation. 28S, 18S and Mds-1 (900 bp) along with arrows on the left of the northern blot represent the locations of 28S rRNA, 18S rRNA andMds-1mRNA. An 18S rRNA image is given as loading control. Interaction phenotypes are given under the 18S rRNA images with: R, resistant; S, susceptible. (b) Heat stress inducesMds-1. Northern blot and phenotypic analyses of resistant genotype Molly seedlings that were either unstressed (20 °C) or stressed at 30 or 35 °C. (c) The decay of heat-inducedMds-1transcript and protein correlates with restoration of Molly resistance to Hessian fly. Northern (upper panel), western (lower panel) and phenotypic analyses on Molly plants were conducted during recovery after stress. Seedlings were stressed at 37 °C for 12 or 24 h, and some 24 h-stressed plants were allowed to recover at 20 °C for 3–48 h. Denotations for northern blot and phenotypic analysis are the same as ina. The positions of protein size markers and the location of the Mds-1 protein are given on the left of the western blot. A coomassie-blue stained gel image is give under the blot as loading control. Plants were infested with Hessian fly biotypeGP. Figure 3: Ectopic expression and heat induction of Mds-1 in resistant wheat. ( a ) Ectopic expression of Mds-1 correlates with a phenotype switch of Molly plants from resistance to susceptibility to Hessian fly biotype GP infestation. Northern blot analysis of Mds-1 transcript in samples from transgenic Molly lines T640, T1166 and T1417 ( Supplementary Table S2 , Supplementary Fig. S9 ); non-transgenic, resistant Molly; and the susceptible wheat Newton with (I) and without (U) Hessian fly (biotype GP ) infestation. 28S, 18S and Mds-1 (900 bp) along with arrows on the left of the northern blot represent the locations of 28S rRNA, 18S rRNA and Mds-1 mRNA. An 18S rRNA image is given as loading control. Interaction phenotypes are given under the 18S rRNA images with: R, resistant; S, susceptible. ( b ) Heat stress induces Mds-1 . Northern blot and phenotypic analyses of resistant genotype Molly seedlings that were either unstressed (20 °C) or stressed at 30 or 35 °C. ( c ) The decay of heat-induced Mds-1 transcript and protein correlates with restoration of Molly resistance to Hessian fly. Northern (upper panel), western (lower panel) and phenotypic analyses on Molly plants were conducted during recovery after stress. Seedlings were stressed at 37 °C for 12 or 24 h, and some 24 h-stressed plants were allowed to recover at 20 °C for 3–48 h. Denotations for northern blot and phenotypic analysis are the same as in a . The positions of protein size markers and the location of the Mds-1 protein are given on the left of the western blot. A coomassie-blue stained gel image is give under the blot as loading control. Plants were infested with Hessian fly biotype GP . 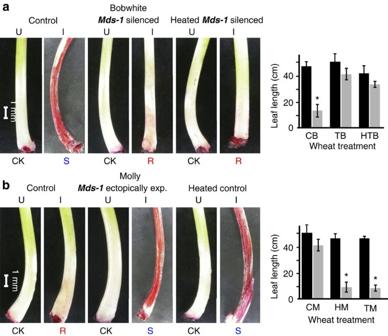Figure 4:Mds-1expression levels affect Hessian fly infestation. Hessian fly biotypeGPwas used for all infestation. (a)Mds-1silencing inhibits Hessian fly-mediated nutritive cell formation and plant-growth suppression. The left panel shows epidermal permeability as indicated by neutral red staining in control,Mds-1-silenced and heat-stressedMds-1-silenced Bobwhite. The letters U and I indicate uninfested and infested plants. Resistant (R) or susceptible (S) phenotypes of infested plants and uninfested controls (CK) are below the images. The right panel shows growth inhibition of cultivar Bobwhite by Hessian fly. Solid bars, uninfested; grey bars, infested plants of control Bobwhite (CB),Mds-1-silenced Bobwhite (TB) or heat-stressed,Mds-1-silenced Bobwhite (HTB). Four replicates were carried out for each analysis. Data were subjected to analysis of variance using ProStat software (Poly Software International Inc., Pearl River, NY, USA). *Indicates significance level atP≤0.05. Standard error is given in each graph. (b) High levels ofMds-1expression in wheat confer avirulent insects (biotypeGP) the ability to manipulate normally resistant Molly plants. The left panel shows neutral red staining of leaf-sheaths.Mds-1-ectopically expression indicates Molly plants withMds-1ectopically expressed. Other denotations are the same as ina. The right panel shows growth inhibition of Molly seedlings by biotypeGP. Solid bars, uninfested; grey bars, infested plants of control Molly (CM), heat-stressed Molly (HM) or Molly withMds-1ectopic expression (TM). Four replicates were carried out for each analysis and standard error is given in the figure. Full size image Figure 4: Mds-1 expression levels affect Hessian fly infestation. Hessian fly biotype GP was used for all infestation. ( a ) Mds-1 silencing inhibits Hessian fly-mediated nutritive cell formation and plant-growth suppression. The left panel shows epidermal permeability as indicated by neutral red staining in control, Mds-1 -silenced and heat-stressed Mds-1 -silenced Bobwhite. The letters U and I indicate uninfested and infested plants. Resistant (R) or susceptible (S) phenotypes of infested plants and uninfested controls (CK) are below the images. The right panel shows growth inhibition of cultivar Bobwhite by Hessian fly. Solid bars, uninfested; grey bars, infested plants of control Bobwhite (CB), Mds-1 -silenced Bobwhite (TB) or heat-stressed, Mds-1 -silenced Bobwhite (HTB). Four replicates were carried out for each analysis. Data were subjected to analysis of variance using ProStat software (Poly Software International Inc., Pearl River, NY, USA). *Indicates significance level at P ≤0.05. Standard error is given in each graph. ( b ) High levels of Mds-1 expression in wheat confer avirulent insects (biotype GP ) the ability to manipulate normally resistant Molly plants. The left panel shows neutral red staining of leaf-sheaths. Mds-1 -ectopically expression indicates Molly plants with Mds-1 ectopically expressed. Other denotations are the same as in a . The right panel shows growth inhibition of Molly seedlings by biotype GP . Solid bars, uninfested; grey bars, infested plants of control Molly (CM), heat-stressed Molly (HM) or Molly with Mds-1 ectopic expression (TM). Four replicates were carried out for each analysis and standard error is given in the figure. Full size image Mds-1 silencing suppresses susceptibility metabolic changes The impact of Mds-1 silencing and ectopic expression on epidermal permeability (an indicator of nutritive cell formation) [4] , plant-growth inhibition and expression of nutrition-related host genes were examined in wheat with or without Hessian fly infestation. Hessian fly infestation induced strong epidermal permeability, as measured by the uptake of neutral red dye, in control Bobwhite ( Fig. 4a ), as compared with background staining of uninfested control Bobwhite ( Fig. 4a1 , UCB). Uninfested, Mds-1 -silenced Bobwhite plants displayed neutral red uptake comparable to untreated control Bobwhite plants, and Hessian fly infestation failed to induce epidermal permeability in Mds-1 -silenced Bobwhite plants. Heat-stress treatment also had no effect on permeability in either uninfested or infected Mds-1 -silenced Bobwhite plants. Mds-1 silencing also prevented the plant-growth inhibition that is observed after Hessian fly infection of control Bobwhite plants (right panel). Heat treatment could not induce susceptibility in the silenced plants either. On the other hand, high levels of ectopic Mds-1 expression allowed the normally avirulent biotype GP to induce strong epidermal permeability in the otherwise resistant wheat cultivar Molly ( Fig. 4b ). High level of Mds-1 expression induced by heat stress also allowed biotype GP to induce strong epidermal permeability of Molly cells. High levels of Mds-1 expression through either heat stress or ectopic expression allowed the normally avirulent Hessian fly biotype to inhibit plant growth. Mds-1 silencing also limited the ability of Hessian fly to upregulate nutrient production-related genes and downregulate defence genes in the susceptible host Bobwhite, a phenomenon normally observed only in resistant plants during incompatible interactions ( Supplementary Fig. S11 ). Mds-1 is correlated with powdery mildew susceptibility To determine whether Mds-1 is specific to Hessian fly or a common susceptibility gene to other biotrophics as well, transgenic plants with Mds-1 silenced were tested against two wheat biotrophic pathogens, the powdery mildew caused by the fungus B. graminis f. sp. tritici ; and the leaf rust caused by the fungus Puccinia triticina . Inoculation of wheat seedlings with the isolate KS-5 of B. graminis f. sp. tritici revealed that all tested transgenic Bobwhite lines with Mds-1 silenced exhibited reduced lesion size in response to the pathogen, whereas control Bobwhite plants displayed full-lesion development that is consistent with susceptibility ( Fig. 5a , Supplementary Table S2 ). B. graminis f. sp. tritici infection strongly upregulated Mds-1 in powdery mildew-susceptible cultivars Molly, Newton and Bobwhite, but only slightly affected Mds-1 transcript abundance in the powdery mildew-resistant cultivar Duster ( Fig. 5b ), which contains the R gene Pm3 (ref. 17 ). Conversely, high levels of Mds-1 transcript in Duster, as induced by heat stress ( Fig. 5c ), were correlated with a phenotype switch from resistant to susceptible to B. graminis f. sp. tritici ( Fig. 5d ). On the other hand, inoculation of wheat seedlings with the PRTUSS4 strain of the rust pathogen Puccinia triticina revealed that Mds-1 silencing does not affect wheat resistance or susceptibility to the rust fungal pathogen ( Supplementary Fig. S12 ). 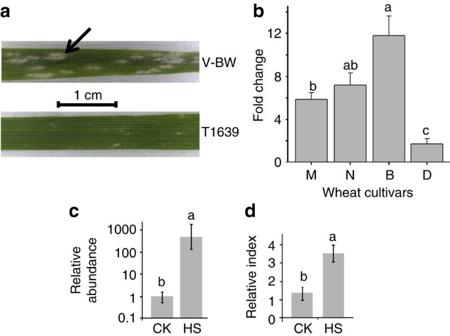Figure 5: Levels ofMds-1expression affect development ofB. graminisf. sp.tritici. (a)Mds-1silencing inhibits virulence ofB. graminisf. sp.triticion the susceptible wheat Bobwhite. Large lesions (arrow) on a vector-transformed, Bobwhite plant (V-BW), small lesions on theMds-1-silenced plant T1639. (b)Mds-1transcript increases followingB. graminisf. sp.triticiinfection in susceptible cultivars Molly (M), Newton (N) and Bobwhite (B), but not in the resistant cultivar Duster (D) based on real-time PCR (qPCR) results of samples 24 h after inoculation. Three biological replicates were carried out for qPCR. Data were subjected to analysis of variance analysis. Tukey’s pairwise comparisons based on Student’s range statistics were then conducted. Tukey’s 95% simultaneous confidence intervals for pair-wise comparisons were used to separate data into groups with significant differences. Lower case letters indicate different groups atP≤0.05. Standard error is given in the figure. (c) Heat stress (HS, at 35 °C for 24 h) inducesMds-1expression over 100 fold in the resistant cultivar Duster compared with control plants (CK) determined by qPCR. Three replicates were carried out and standard error is given in the figure. (d) HS compromises the resistance of Duster toB. graminisf. sp.tritici. The relative disease index was 1.3±0.5 on control plants (CK), but climbed to 3.6±0.4 on plants stressed at 35 °C for 24 h (HS) on a scale of 0–4. Figure 5: Levels of Mds-1 expression affect development of B. graminis f. sp. tritici . ( a ) Mds-1 silencing inhibits virulence of B. graminis f. sp. tritici on the susceptible wheat Bobwhite. Large lesions (arrow) on a vector-transformed, Bobwhite plant (V-BW), small lesions on the Mds-1 -silenced plant T1639. ( b ) Mds-1 transcript increases following B. graminis f. sp. tritici infection in susceptible cultivars Molly (M), Newton (N) and Bobwhite (B), but not in the resistant cultivar Duster (D) based on real-time PCR (qPCR) results of samples 24 h after inoculation. Three biological replicates were carried out for qPCR. Data were subjected to analysis of variance analysis. Tukey’s pairwise comparisons based on Student’s range statistics were then conducted. Tukey’s 95% simultaneous confidence intervals for pair-wise comparisons were used to separate data into groups with significant differences. Lower case letters indicate different groups at P ≤0.05. Standard error is given in the figure. ( c ) Heat stress (HS, at 35 °C for 24 h) induces Mds-1 expression over 100 fold in the resistant cultivar Duster compared with control plants (CK) determined by qPCR. Three replicates were carried out and standard error is given in the figure. ( d ) HS compromises the resistance of Duster to B. graminis f. sp. tritici . The relative disease index was 1.3±0.5 on control plants (CK), but climbed to 3.6±0.4 on plants stressed at 35 °C for 24 h (HS) on a scale of 0–4. Full size image Our data with RNAi suppression and ectopic expression of Mds-1 indicate that Mds-1 is sufficient to confer wheat susceptibility to Hessian fly infestation. However, the susceptibility of Chinese Spring deletion lines lacking Mds-1 or one of its homoeologs on 3BS and 3DS suggests that both Mds-1 and its homoeologs can confer wheat susceptibility to Hessian fly. This is not surprising considering the fact that diploid goatgrass (with D genome only) is also a host of Hessian fly, and the fact that the coding sequences of Mds-1 and its the homoeologs are highly conserved ( Supplementary Fig. S8 ). Interestingly, the promoter and 3′ non-coding regions are highly diversified among Mds-1 and related genes. The difference in the promoter and non-coding regions is consistent with significant variation in the expression levels among Mds-1 homoeologous genes in response to Hessian fly infestation and heat stress ( Supplementary Fig. S7 ) [5] . Therefore, the functions of these highly conserved proteins may be differentiated through differential expression under different conditions. Mds-1 is among the most induced by Hessian fly infestation as well as under heat stress ( Supplementary Figs S5 and S7 ) [5] , suggesting its involvement in wheat susceptibility to Hessian fly in the wheat lines we studied. Indeed, Mds-1 is sufficient for inducing a state of susceptibility as evidenced by the conversion of the resistant cultivar Molly to susceptibility by ectopic expression of Mds-1 alone in multiple independent transgenic lines. The mechanism for Mds-1 in wheat susceptibility remains to be determined. The inability of Hessian fly larvae to induce Mds-1 in the presence of an effective R gene suggests that the R protein blocks Mds-1 induction by virulent effectors from Hessian fly ( Fig. 6 ). The conversion of resistant plants into susceptibility under the condition of high levels of Mds-1 expression suggests that MDS-1 either suppresses plant defences, activates susceptibility pathways, or a combination of both. Our data points to the possibility that MDS-1 suppresses host defence as suggested by the upregulation of defence genes in plants with an effective R gene and in Mds-1 -silenced transgenic plants ( Supplementary Fig. S11 ), and activates susceptibility pathways as indicated by upregulation of nutrient metabolic pathways and the formation of nutritive cells ( Fig. 4 , Supplementary Fig. S11 ). During compatible interactions, Mds-1 is likely induced by Hessian fly or fungal effectors through interactions with Mds-1 regulatory elements directly or indirectly [18] , or pathways that lead to activation of heat-shock transcription factors ( Fig. 6 ) [19] , [20] , [21] . The MDS-1 protein may then suppress plant defences, and activate, directly or indirectly, wheat susceptibility pathways, or serve as a component to allow effectors from Hessian fly and B. graminis f. sp. tritici to activate wheat susceptibility pathways. The activation of wheat susceptibility pathways leads to metabolic changes in the host [5] , [10] , resulting, in the case of Hessian fly, in the formation of nutritive cells and plant susceptibility [3] . During incompatible interactions, the prevention of Mds-1 induction by Hessian fly due to an intervention from a specific R–AVR protein recognition inhibits the induction of Mds-1 and thus nutritive cell formation. The lack of nutrients and the activation of defence pathways result in plant resistance. 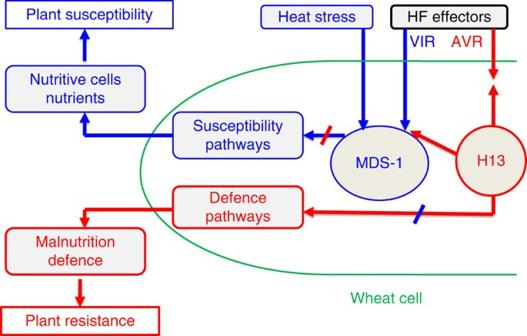Figure 6: A model forMds-1involvement in plant susceptibility. Blue arrows between objects indicate conditions leading to plant susceptibility throughMds-1upregulation. Red arrows between objects indicate conditions leading to plant resistance through the prevention ofMds-1induction. The arrows between MDS-1 and H13 R protein indicate possible interactions between them. During compatible interactions in susceptible plants, virulent (VIR) effectors from Hessian fly upregulateMds-1expression either directly by targetingMds-1regulatory elements or indirectly through activating heat-shock transcription factor(s). High levels ofMds-1expression result in activation of susceptibility pathways, leading to the reprogramming of metabolic pathways, suppression of plant defence, and the formation of nutritive cells at the feeding site of host plants. During incompatible interactions in plants with R geneH13, the corresponding Avirulence (AVR) effector from Hessian fly is recognized by H13 R protein, leading to blockage ofMds-1upregulation and activation of defence pathways. The suppression of high levelMds-1expression inhibit nutritive cell formation and possibly other susceptibility events, leading to Hessian fly larval death due to the lack of nutrition and possibly increased toxicity. Figure 6: A model for Mds-1 involvement in plant susceptibility. Blue arrows between objects indicate conditions leading to plant susceptibility through Mds-1 upregulation. Red arrows between objects indicate conditions leading to plant resistance through the prevention of Mds-1 induction. The arrows between MDS-1 and H13 R protein indicate possible interactions between them. During compatible interactions in susceptible plants, virulent (VIR) effectors from Hessian fly upregulate Mds-1 expression either directly by targeting Mds-1 regulatory elements or indirectly through activating heat-shock transcription factor(s). High levels of Mds-1 expression result in activation of susceptibility pathways, leading to the reprogramming of metabolic pathways, suppression of plant defence, and the formation of nutritive cells at the feeding site of host plants. During incompatible interactions in plants with R gene H13 , the corresponding Avirulence (AVR) effector from Hessian fly is recognized by H13 R protein, leading to blockage of Mds-1 upregulation and activation of defence pathways. The suppression of high level Mds-1 expression inhibit nutritive cell formation and possibly other susceptibility events, leading to Hessian fly larval death due to the lack of nutrition and possibly increased toxicity. Full size image Hessian fly induces cells in the wheat sheath to develop into nutritive cells for the nourishment of fly larvae, which involves the conversion of host sheath cells to a nutritional sink. The process also induces a variety of stress-related genes, which initially were construed to reflect the host response to infection. However, the evidence presented here indicates that the Hessian fly specifically exploits the HSP gene Mds-1 and other related genes for the benefit of larval growth. Our results adds another dimension to the remarkable and ancient small HSP family proteins, including MDS-1, which are involved in a wide range of functions from construction of the animal eye lens to stress responses [22] . The proliferation of small HSP genes in plants has been postulated to be an adaptation to dynamic environmental changes, including heat stress. Our results indicate that the Hessian fly and B. graminis f. sp. tritici exploit a heat shock-like response that leads to host susceptibility. Remarkably, the Mds-1- silenced plants were observed to be poor hosts for the powdery mildew fungus B. graminis f. sp. tritici . Measurements of Mds-1 expression during infection of normal wheat plants revealed that Mds-1 is also induced to higher levels of expression during B. graminis infection. The wheat variety Duster is resistant to many strains of B. graminis f. sp. tritici , including the KS-5 isolate, and very low Mds-1 expression was detected in Duster plants challenged by the fungus. Ectopic expression studies of Mds -1 were not conducted in the Duster variety. Nonetheless, heat stress of Duster led to both elevated levels of Mds-1 and the loss of resistance. The possibility exists that B. graminis f. sp. tritici specifically exploits the heat-shock pathway to suppress host immunity responses. The effect of Mds-1 silencing on susceptibility, however, did not extend to the leaf rust pathogen Puccinia triticina as silenced plants were equally susceptible to rust infection as normal plants ( Supplementary Fig. S12 ). The possible negative impact of Mds-1 silencing on wheat remains to be determined. Initial examination of apparent phenotypic abnormalities in Mds-1 -silenced wheat lines include partial sterility, smaller grain weight, reduced plant height and low seed germination rates ( Supplementary Table S4 ). However, abnormalities in plants with Mds-1 silenced vary from plant to plant and may have been caused by positional effects due to different integration sites of the Mds-1 construct into the wheat genome or by tissue culture. For practical application, potential negative impact needs to be eliminated or reduced to minimum for economic benefit. One way to reduce potential negative impact is to use tissue-specific promoters for gene silencing [23] . The rice S gene, Pi21 , which encodes a transporter-like protein and is highly conserved among monocots, has been engineered for broad resistance to rice blast [24] . Unlike R genes that have similar structures and possibly similar action modes [25] , S genes exhibit greater variations in structures and functional mechanisms [26] , [27] , [28] , [29] , [30] . The variation in S genes provides us opportunities for fundamental research to reveal mechanisms of plant susceptibility and resistance, as well as for practical applications to develop plants with improved resistance for pest management. The effect of Mds-1 expression in wheat on resistance to Hessian fly and the loss of resistance to both Hessian fly and powdery mildew upon heat stress also provided insight into the resistance mechanisms. Numerous plant species with single major R genes lose resistance to herbivores under heat stress, suggesting a possible role of Hsp genes in plant susceptibility [9] , [31] , [32] , [33] , [34] . The observations that a bacterial pathogen injects an HSP-like protein into host cells for virulence, and elevation in HSP70 levels induced by heat stress makes plants susceptible to an otherwise avirulent pathogen also support a role of HSPs in plant susceptibility [35] . However, various HSPs including HSP90, HSP70, an HSP-like protein, and a small HSP have been found to interact with disease resistance protein complexes and are required for disease resistance [36] , [37] , [38] , [39] , [40] , [41] , [42] , [43] . The basis for the role of MDS-1 and possibly other HSPs as well in plant susceptibility and the role of HSPs in plant resistance remains to be revealed. In a similar situation, receptor-like kinase genes are required for both fungal susceptibility and resistance in different plant–pathogen systems [26] , [27] . The dominant effect of Mds-1 and possibly other temperature-dependent susceptibility genes under elevated temperatures pose a threat to the effectiveness of plant resistance to Hessian fly and other pests under scenarios of global climate change [32] , [44] , [45] , [46] . A better understanding of the molecular mechanisms of Mds-1 and other temperature-dependent, dominant susceptibility genes is needed to preserve plant resistance in the face of global warming. Wheat ( Triticum aestivum ) genotypes Bobwhite is a spring wheat cultivar susceptible to Hessian fly and powdery mildew ( B. graminis f. sp. tritici ). Bobwhite is widely used for producing transgenic plants because of its high efficiency for genetic transformation, and was used for generating RNAi transgenic plants. Newton, a winter wheat with no Hessian fly R gene, was used as susceptible control. Molly and Iris, two near-isogenic lines of Newton, contain H13 and H9 R genes, respectively [12] . WGRC42 contains R gene Hdic (ref. 47 ). Duster is powdery mildew resistant with R gene Pm3c (ref. 17 ). Seedlings were grown in pots, 10 cm in diameter, in Pro-Mix ‘BX’ medium (Hummert, Topeka, KS) in growth chambers (Model AR-66L, Percival, Perry, IA) with a 16/8 h light/dark cycle at 275 μmol m −2 s −1 under 20/18 °C day/night. Heat stress was delivered by adjusting temperature with other conditions unchanged. Infestation and sample collection Hessian fly biotypes: GP avirulent to all known resistance (R) genes, vH9 virulent to H9 , vH13 virulent to H13 (refs 48 , 49 ). Hessian fly populations with mixed biotypes were also used ( Supplementary Table S1 ) [50] . Wheat seedlings were infested with ~15 eggs/plant by confining flies with a mesh screen cage. The time when neonates just reached the feeding site was taken as the initial infestation time (monitored by dissecting extra infested plants). Wheat tissues were collected 12–96 h later from the initial infestation time. Plants were phenotyped 2 weeks later with resistance defined as normal wheat growth and insect death, and susceptibility defined as stunted wheat growth and normal insect development. Leaf-sheath tissue of 10–15 mm at the feeding site was cut out, insects removed and used for various analyses. Each sample contained a pool of 10 plant tissues. Samples were frozen immediately in liquid nitrogen and stored at −80 °C. Powdery mildew Isolate KS-5 of B. graminis was used for infection. A conidia suspension was uniformly sprayed onto plants, and the plants were placed in a chamber for symptom development. Phenotype was scored 8 days post inoculation. Disease evaluation was based on a 0–4 scale as described previously [51] . DNA and RNA extraction and blot analysis Genomic DNA was extracted from wheat tissues following CTAB procedure [47] . Plasmid DNA was extracted using a QIAprep Miniprep Kit (Qiagen). Total RNA was extracted using TRI reagent (Molecular Research Inc., Cincinnati, OH). RNA samples were further purified through an RNease kit (Qiagen). DNA and RNA were quantified with a NanoDrop-1000. Northern blot analysis was carried out as described previously [5] . Mds-1 cloning On the basis of EST sequence, a full cDNA was cloned using a SMART RACE Kit (Clontech, Mountain View, CA) with primers in Supplementary Table S3 . The RACE-PCR product was gel-purified using a GeneClean Turbo for PCR Kit (Qbiogene, Carlsbad, CA), and cloned directly into the vector pCR II-TOPO (Qbiogene). Positive clones were sequenced using M13 primers contained in the vector. Full-length Mds-1 gene was cloned by PCR with DNA from Newton using primers Mds-1Lb and Mds-1R ( Supplementary Table S3 ). Sequence alignments were produced using ClustalW2 (ref. 52 ) and printed using BoxShade. Western blot analysis A full-length recombinant protein was produced and used for a polyclonal antibody in rabbits by GenScript (Piscataway, NJ). The antibody was affinity purified. Protein extracts were prepared by homogenizing wheat tissues in Tris–HCl buffer (pH 8.0) containing protease inhibitor cocktail (Sigma, St Louis, MO). Protein concentration was measured using a bicinchoninic acid kit (Sigma). About 180 μg of protein extract was loaded onto a 12% gel and separated using Xcell surelock electrophoresis cell (Invitrogen, Carlsbad, CA ). Proteins were transferred to PVDF membrane (Millipore, Danvers, MA). The membrane was blocked using 5% (w/v) milk in Tris-buffered Saline (100 mM Tris, pH7.4, 150 mM NaCl) with 0.1% Tween 20 (TBST) for 1 h at 4 °C. The membrane was then incubated overnight at 4 °C with primary antibody–horseradish peroxidase conjugation (0.5 μg ml −1 of 2% milk/TBST). The membrane was then washed three times in TBST and incubated for 1 min with horseradish peroxidase chemiluminescent detection reagents (Invitrogen). The membrane was exposed to film for 4 h before development. VIGS treatment Barley stripe mosaic virus (BSMV) [53] was used for VIGS [13] , [54] , [55] . A 338 bp 3′-fragment of Mds-1 was amplified by PCR with primers Mds-1La and Mds-1R ( Supplementary Table S3 ). The PCR fragment was ligated into the γ-genome at antisense orientation. Infectious RNA transcripts were synthesized using a mMessage mMachine T7 transcription kit (Ambion, Austin, TX) from linearized α, β and γ target plasmids [13] . The silencing BSMV inoculum was made by combining an equal molar ratio of α, β and γ transcripts with excess inoculation buffer containing a wounding agent (FES). The first leaf of 10-day-old seedlings was inoculated and plants were then infested with Hessian fly after apparent visual symptom 8 days post-BSMV inoculation. Mds-1 knockdown construct An RNAi-based construct was made according to the Gateway system (Invitrogen). The 338-bp Mds-1 fragment was amplified as in VGIS. PCR product was directionally inserted into pENTR/ D-TOPO. The final RNAi construct was made by recombination from an LR clonase reaction using a Gateway LR clonase enzyme mix between the entry vector carrying the Mds-1 fragment and the pANDA-mini vector [56] , from which the identical Mds-1 fragment was inserted into both sides of the 920-bp GUS linker in antisense and sense orientations. The transcribed RNA contains a hairpin that forms dsRNA. Mds-1 expression construct Full Mds-1 -coding region was amplified by PCR with primers Mds-1Lc and Mds-1R ( Supplementary Table S3 ). Mds-1Lc contains the start codon and an added sequence with a BCL I restriction site (5′-TGATCA-3′). An internal BCL I site exists in the 3'-UTR. PCR product was digested with BCL I, and the resulting DNA fragment was ligated into pAHC17 at the Bam HI site [57] . The resulting construct contains full Mds-1 -coding region under a maize ubiquitin promoter ( Ubi-1 ). Transgenic plants For silencing, the pANDA construct and pAHC20 containing the bar gene were co-bombarded with 1:1 ratio into embryogenic calli as described by Altpeter [58] and modified by Ayella et al . [56] Briefly, embryos (2–5 mm) were then excised from immature seeds and plated on CM4 media to initiate the formation of somatic embryo for 2–7 days. Somatic embryos were selected for highly embryogenic calli and were co-bombarded with pAHC20 and GOI plasmids at 1:1 ratio by using the particle inflow gun. After 5 days wheat calli were placed on CM4 medium containing 5 mg l −1 glufosinate for 2 weeks. Cultures were transferred twice to CM4 medium with 10 mg l −1 glufosinate for 2 weeks each. The growing embryogenic tissues were transferred to shoot production medium (MSP) with 5 mg l −1 glufosinate selection until green shoots were observed. The cultures were then retransferred to elongation and rooting medium (MSE) containing 5 mg l −1 glufosinate but not 2,4-D for 2–3 weeks. Shoots that developed roots were then transferred to potting soil. Recovered plants were screened for herbicide resistance with 0.2% Liberty (AgEvo, Pikeville, NC). Plants survived are presumably transformed with pAHC20, which usually indicates a high probability of cotransformation with the target construct. Herbicide-resistant plants were analysed for Mds-1 construct presence with PCR. Epidermal permeability Neutral red stain (Sigma, St Louis, MO) was used to determine epidermal permeability as described [4] . Real-time PCR Quantitative PCR was performed as described previously [59] . Primers were designed using the software package Beacon Designer 7 ( Supplementary Table S3 ). RNA was collected from three biological replicates. Relative fold-changes for transcripts were calculated using the comparative 2 −ΔΔCT method [60] and normalized to actin control. Statistical test Three biological replicates were carried out for each quantitative PCR analysis. Data were subjected to analysis of variance, and Tukey’s honestly significant difference multiple comparisons were conducted using ProStat software Version 5.5(Poly Software International Inc., Pearl River, NY, USA). Tukey’s 95% simultaneous confidence intervals were used to separate data into groups. The lower case letters were used to represent different groups with statistically significant difference at P ≤0.05. Accession Codes The sequence for Mds-1 has been deposited in the NCBI Nucleotide database under accession code JN162442. How to cite this article: Liu, X. et al . Wheat Mds-1 encodes a heat-shock protein and governs susceptibility towards the Hessian fly gall midge. Nat. Commun. 4:2070 doi: 10.1038/ncomms3070 (2013).